Substrate docking to γ-secretase allows access of γ-secretase modulators to an allosteric site γ-Secretase generates the peptides of Alzheimer's disease, Aβ 40 and Aβ 42 , by cleaving the amyloid precursor protein within its transmembrane domain. γ-Secretase also cleaves numerous other substrates, raising concerns about γ-secretase inhibitor off-target effects. Another important class of drugs, γ-secretase modulators, alter the cleavage site of γ-secretase on amyloid precursor protein, changing the Aβ 42 /Aβ 40 ratio, and are thus a promising therapeutic approach for Alzheimer's disease. However, the target for γ-secretase modulators is uncertain, with some data suggesting that they function on γ-secretase, whereas others support their binding to the amyloid precursor. In this paper we address this controversy by using a fluorescence resonance energy transfer-based assay to examine whether γ-secretase modulators alter Presenilin-1/γ-secretase conformation in intact cells in the absence of its natural substrates such as amyloid precursor protein and Notch. We report that the γ-secretase allosteric site is located within the γ-secretase complex, but substrate docking is needed for γ-secretase modulators to access this site. Presenilin-1 (PS1)/γ-secretase is responsible for the final cut of the amyloid precursor protein (APP) to generate the Aβ peptide [1] , [2] . The two major Aβ species, Aβ 40 and Aβ 42 , are produced in an approximately 9:1 ratio. The longer Aβ 42 peptide is more prone to forming toxic oligomeric species, and is believed to be involved in the pathogenesis of Alzheimer's disease (AD) [3] , [4] . Because γ-secretase cleaves other essential proteins (for example, the Notch receptor), simple γ-secretase inhibition raises concern for off-target effect. Another important class of drugs, γ-secretase modulators (GSMs), alter the cleavage site of γ-secretase on APP, changing the Aβ 42 / 40 ratio [5] , [6] , [7] , [8] , and are thus a promising therapeutic approach for AD. We have previously reported that alterations in the Aβ 42/40 ratio are tightly linked to conformational changes in PS1 [9] , [10] , [11] . To analyse conformational change in PS1 in living cells, we have recently developed the G-PS1-R fluorescent probe, which has green fluorescent protein (GFP) at the PS1 N terminus (NT) and RFP in the large cytosolic-loop domain ( Fig. 1a ). This enables us to monitor PS1 conformation (that is, PS1 NT to loop proximity) by FRET/fluorescent lifetime imaging microscopy (FLIM). Using this probe, we demonstrated that FRET reflects PS1 conformation, reliably predicting the Aβ 42/40 ratio. We found that PS1 adopts a 'closed' conformation (that is, close PS1 NT-loop proximity) in response to various manipulations that increase the Aβ 42/40 ratio (for example, fenofibrate treatment, familial Alzheimer's disease (FAD) PS1 mutations and Pen-2 NT modification), whereas the 'open' conformation (greater distance between the PS1 NT and loop) corresponds to a lower Aβ 42/40 ratio (for example, in response to ibuprofen treatment) [11] . 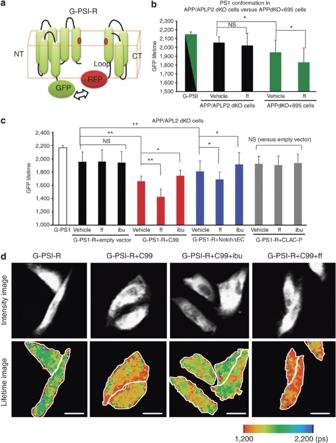Figure 1: Substrate-dependent and -independent changes of PS1 conformation. (a) Schematic structure of the G-PS1-R probe. GFP is fused to the PS1 N terminus (NT), and RFP is inserted into the large cytoplasmic loop between transmembrane domains 6 and 7. The red dots indicate D257 and D385 catalytic site aspartates. (b) FLIM analysis of the PS1 conformation in APP/APLP2 dKO cells (black bars) and in APP/APLP dKO cells reconstituted by stable expression of APP695 (APPdKO+695, green bars). GFP-PS1 (G-PS1)-transfected cells were used as a negative control to establish GFP lifetime in the absence of an acceptor fluorophore, which was comparable in APP/APLP2 dKO and APPdKO+695 cells (black and green bars, respectively). The GFP lifetime in G-PS1-R-transfected cells was compared in APP/APLP dKO and APP/APLP dKO+695 cells treated with vehicle or fenofibrate (ff) in three independent experiments (mean±s.d.; *P<0.001; NS, not significant; Fisher's PSLD, ANOVA;n=15–18 cells per condition were examined). (c) PS1 conformation was monitored in APP/APLP2 dKO cells co-transfected with G-PS1-R probe and either empty vector (black bars), C99 (red bars), NotchΔEC (blue bars) or CLAC-P (grey bars) constructs. The cells were treated with vehicle control, 100 μM fenofibrate (ff) or 400 μM ibuprofen (ibu) for 24 h. The graph shows mean±s.d. lifetime in psec; *P<0.05, **P<0.001; NS, not significant; ANOVA,n=3–5 independent experiments. On an average, 12–33 (vehicle), 17–20 (ff) and 12–18 (ibu) cells were examined. (d) The intensity images show GFP fluorescence reflecting the expression pattern of G-PS1-R probe. Pseudo-coloured FLIM images show subcellular distribution of the GFP lifetimes, with red pixels representing shorter lifetime (closer GFP-PS1 NT and RFP-PS1-loop proximity). Expression of the C99 substrate significantly increases red pixels, especially at the cell periphery. Ibuprofen reduces and fenofibrate increases the amount of red pixels, indicating 'opening' and 'closing' of the G-PS1-R conformation, respectively. The cell profiles are shown by tracing. A colourimetric scale bar shows colour-coded fluorescence lifetime in picoseconds. Figure 1: Substrate-dependent and -independent changes of PS1 conformation. ( a ) Schematic structure of the G-PS1-R probe. GFP is fused to the PS1 N terminus (NT), and RFP is inserted into the large cytoplasmic loop between transmembrane domains 6 and 7. The red dots indicate D257 and D385 catalytic site aspartates. ( b ) FLIM analysis of the PS1 conformation in APP/APLP2 dKO cells (black bars) and in APP/APLP dKO cells reconstituted by stable expression of APP695 (APPdKO+695, green bars). GFP-PS1 (G-PS1)-transfected cells were used as a negative control to establish GFP lifetime in the absence of an acceptor fluorophore, which was comparable in APP/APLP2 dKO and APPdKO+695 cells (black and green bars, respectively). The GFP lifetime in G-PS1-R-transfected cells was compared in APP/APLP dKO and APP/APLP dKO+695 cells treated with vehicle or fenofibrate (ff) in three independent experiments (mean±s.d. ; * P <0.001; NS, not significant; Fisher's PSLD, ANOVA; n =15–18 cells per condition were examined). ( c ) PS1 conformation was monitored in APP/APLP2 dKO cells co-transfected with G-PS1-R probe and either empty vector (black bars), C99 (red bars), NotchΔEC (blue bars) or CLAC-P (grey bars) constructs. The cells were treated with vehicle control, 100 μM fenofibrate (ff) or 400 μM ibuprofen (ibu) for 24 h. The graph shows mean±s.d. lifetime in psec; * P <0.05, ** P <0.001; NS, not significant; ANOVA, n =3–5 independent experiments. On an average, 12–33 (vehicle), 17–20 (ff) and 12–18 (ibu) cells were examined. ( d ) The intensity images show GFP fluorescence reflecting the expression pattern of G-PS1-R probe. Pseudo-coloured FLIM images show subcellular distribution of the GFP lifetimes, with red pixels representing shorter lifetime (closer GFP-PS1 NT and RFP-PS1-loop proximity). Expression of the C99 substrate significantly increases red pixels, especially at the cell periphery. Ibuprofen reduces and fenofibrate increases the amount of red pixels, indicating 'opening' and 'closing' of the G-PS1-R conformation, respectively. The cell profiles are shown by tracing. A colourimetric scale bar shows colour-coded fluorescence lifetime in picoseconds. Full size image On the basis of the above findings, we postulated that GSMs function on a yet unidentified 'allosteric site' to shift PS1/γ-secretase conformation into either the 'open' or 'closed' state, which leads to a changed alignment of the γ-secretase with the APP substrate, thereby resulting in a decrease or increase in the Aβ 42/40 ratio, respectively. The presence of this 'allosteric site' within PS1/γ-secretase itself has been suggested in several studies [5] , [6] , [7] . However, it has recently been reported that a subset of biotinylated photoactivatable forms of certain GSMs (that is, fenofibrate, flurbiprofen) could directly label the γ-secretase substrate, APP and to a lesser extent Notch, rather than the components of the γ-secretase complex itself [8] . To address this controversy directly, we examined whether GSMs alter PS1/γ-secretase conformation in the absence of its natural substrates (APP, C99, NotchΔEC) in intact and/or live cells. Treatment with GSMs led to a robust change in γ-secretase conformation only in the presence of substrates or a small helical peptide (HP) docking site inhibitor [12] . The HP shares sequence with the APP transmembrane domain but lacks the previously reported GSM binding site [12] . These data suggest that GSMs affect PS1/γ-secretase conformation by binding to an allosteric site uncovered by occupancy of the enzyme's docking site. We also directly manipulated potential sites of allosteric modulation of the γ-secretase complex [10] , [13] , and found analogous changes in the absence of APP substrate. These findings suggest that the γ-secretase allosteric site is located within the γ-secretase complex itself but substrate docking is needed for GSMs to access this site. The effect of GSMs on PS1 conformation is substrate dependent We used cells lacking APP and APLP2 (APP/APLP2 dKO cells) and expressing undetectable levels of endogenous Notch to dissect the impact of substrate expression on the action of GSMs. First, the proximity between GFP-PS1 NT and RFP-PS1-loop was analysed by FLIM in either APP/APLP2 dKO cells or APP/APLP2 dKO cells reconstituted by stably expressing the human APP695 isoform (APP/APLP2 dKO+695 cells) transfected with the G-PS1-R probe. We found that the GFP donor lifetime was significantly shorter in APP/APLP2 dKO+695 cells, compared with that in APP/APLP2 dKO cells ( Fig. 1b ), indicating closer PS1 NT-loop proximity in the presence of APP substrate. Transient transfection of the full-length (FL) human APP into APP/APLP2 dKO cells led to a similar change in the PS1 conformation ( Supplementary Fig. S1 ). To further validate these findings, we assessed the effect of immediate γ-secretase substrates on PS1 conformation by transient expression of APP C99 and NotchΔEC in APP/APLP2 dKO cells. Similar to FL APP, both C99 and NotchΔEC expression induced significant shortening of the GFP donor lifetime in the G-PS1-R probe ( Fig. 1c ). It has been shown that the PS1 protein, as it matures and trafficks through the secretory pathway, adopts a ring-like structure [14] , [15] , [16] with PS1 N- and C-termini close enough to support FRET [10] . Our current findings suggest that substrate recruitment and/or entry into the γ-secretase induces PS1 conformation change by bringing PS1 NT and loop domains closer together. Next, we asked whether substrate expression is required for GSMs to induce an allosteric conformational change in PS1. We reasoned that if GSMs are primarily targeting APP substrate 8 , they should have little or no effect on PS1 conformation in the absence of APP. Either APP/APLP2 dKO cells or APP/APLP2 dKO+695 cells transfected with the G-PS1-R probe were treated with the Aβ 42 -raising GSM, fenofibrate, to test whether it can induce a 'closed' conformation of PS1. Interestingly, although fenofibrate treatment shortened the lifetime of the GFP donor in APP/APLP2 dKO+695 cells, it failed to induce any conformational change of G-PS1-R in APP/APLP2 dKO cells ( Fig. 1b ). Fenofibrate treatment similarly induced a 'closed' PS1 conformation in APP/APLP2 dKO cells transiently transfected with FL APP ( Supplementary Fig. S1 ). This suggested that the effect of fenofibrate to induce the 'closed' conformation of PS1 is correlated with the presence of APP substrate. 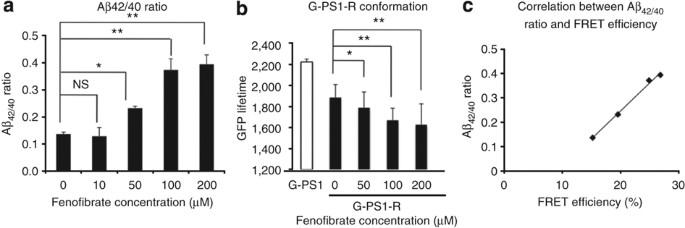Figure 2: Changes in G-PS1-R conformation correlate with changes in the Aβ42/40ratio. CHO cells stably expressing APP (7W cells) were transiently transfected with G-PS1-R probe and treated with the designated concentration of fenofibrate for 24 h. Conditioned media were subjected to Aβ ELISA (a), and the cells were used for the FLIM analysis of GFP lifetimes (G-PS1-R conformation,b). Fenofibrate treatment dose-dependently increased the Aβ42/40ratio (a), and shortened GFP donor lifetime (b). The graph shows mean±s.d.; *P<0.05, **P<0.001; NS, not significant; ANOVA,n=3 independent experiments. (c) FRET efficiency was calculated using the following equation:E%=100*(t1−t2)/t1, wheret1 is G-PS1 lifetime (FRET negative control, no acceptor) andt2 is a second, shorter GFP lifetime in G-PS1-R-transfected cells.E% is plotted against the Aβ42/40ratio. The correlation coefficient=0.99678648 (regression line:y=0.023x−0.2127). Figure 2 shows that fenofibrate increased the Aβ 42/40 ratio ( Fig. 2a ) and altered G-PS1-R conformation ( Fig. 2b ) in a dose-dependent manner in 7W Chinese hamster ovary (CHO) cells stably expressing human FL APP [17] . Figure 2: Changes in G-PS1-R conformation correlate with changes in the Aβ 42/40 ratio. CHO cells stably expressing APP (7W cells) were transiently transfected with G-PS1-R probe and treated with the designated concentration of fenofibrate for 24 h. Conditioned media were subjected to Aβ ELISA ( a ), and the cells were used for the FLIM analysis of GFP lifetimes (G-PS1-R conformation, b ). Fenofibrate treatment dose-dependently increased the Aβ 42/40 ratio ( a ), and shortened GFP donor lifetime ( b ). The graph shows mean±s.d. ; * P <0.05, ** P <0.001; NS, not significant; ANOVA, n =3 independent experiments. ( c ) FRET efficiency was calculated using the following equation: E %=100*( t 1− t 2)/ t 1, where t 1 is G-PS1 lifetime (FRET negative control, no acceptor) and t 2 is a second, shorter GFP lifetime in G-PS1-R-transfected cells. E % is plotted against the Aβ 42/40 ratio. The correlation coefficient=0.99678648 (regression line: y =0.023 x −0.2127). Full size image To explore whether FL APP is needed for the effect of GSMs or if APP C99 will suffice, APP/APLP2 dKO cells were transiently co-transfected with C99 and the G-PS1-R probe and were treated with modulators of the Aβ 42/40 ratio. Similar to the above observations, treatment of C99-expressing cells with fenofibrate also induced a 'closing' of the PS1 conformation, whereas ibuprofen treatment, known to lower the A 42/40 ratio 18 , led to an 'opening' of the G-PS1-R conformation, compared with vehicle-treated cells. This supports the idea that the presence of the immediate γ-secretase substrate is required for the action of these GSMs ( Fig. 1c ). The pseudo-colour FLIM images in Figure 1d show GFP lifetime distribution in APP/APLP2 dKO cells expressing C99 and treated with GSMs. Treatment with aspirin or naproxen, non-steroidal anti-inflammatory drugs (NSAIDs) that do not affect the Aβ 42/40 ratio [18] , had no effect on G-PS1-R conformation in APP/APLP2 dKO cells expressing C99. However, the other two NSAIDs known to modify the Aβ 42/40 ratio, flurbiprofen and celecoxib [19] , had an effect on G-PS1-R conformation, which is comparable to that of ibuprofen and fenofibrate, respectively ( Supplementary Fig. S2 ). Similar to C99, transfection with NotchΔEC facilitated the effect of fenofibrate and ibuprofen on conformational changes of the G-PS1-R protein in APP/APLP2 dKO cells ( Fig. 1c ). On the contrary, GSMs failed to affect G-PS1-R conformation in the presence of CLAC-P, a type II transmembrane protein that is not a γ-secretase substrate [20] ( Fig. 1c ). This suggests that substrate binding to the PS1/γ-secretase is necessary for the action of GSMs. HP enables GSMs to change PS1 conformation According to Kukar et al ., [8] the APP transmembrane region Aβ29-36 (GAIIGLMV) is the binding site for these GSMs. To determine whether substrate binding of GSMs is necessary for the induction of PS1 conformation change, we took advantage of the previously reported HP γ-secretase docking-site inhibitor [12] , which lacks this putative GSM binding site as well as the APP luminal and cytoplasmic domains ( Fig. 3a ). Surprisingly, both fenofibrate and ibuprofen could modulate PS1 conformation in APP/APLP dKO cells in the presence of HP ( Fig. 3b ). The ability of HP to inhibit APP cleavage by PS1/γ-secretase and APP–PS1 interaction was demonstrated by western blot and FLIM experiments, respectively ( Supplementary Fig. S3a,b ). To test whether ibuprofen and fenofibrate may affect HP binding to the initial substrate-docking site in intact cells, CHO 7W cells or primary neurons were treated with HP in the presence or absence of a GSM, and APP/γ-secretase interactions were monitored by both western blot and FLIM analyses. We reasoned that if a GSM affects HP binding to the initial substrate-docking site, it would interfere with the ability of HP to inhibit APP substrate binding to and processing by γ-secretase. Thus, we monitored the APP substrate binding to γ-secretase by FLIM APP–PS1 proximity assay, and APP cleavage by western blot analysis of the APP C-terminal fragment levels. We did not detect any significant change in the ability of HP to bind to PS1/γ-secretase, and therefore to prevent APP/γ-secretase interactions after treatment with these GSMs ( Supplementary Fig. S3c,d ). 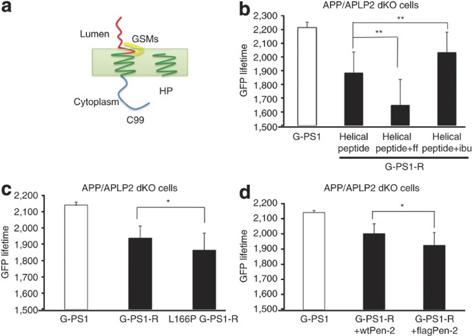Figure 3: FLIM analysis of the changes in GFP-PS1-RFP conformation in APP/APLP2 dKO cells. (a) Schematic representation of the helical peptide, HP and GSM binding site on APP C99. (b) GSMs affect PS1 conformation (NT-loop proximity) in the presence of HP. APP/APLP dKO cells transfected with G-PS1-R probe were treated with either HP alone or HP together with fenofibrate (ff) or ibuprofen (ibu). The graph shows mean±s.d. lifetime in picoseconds; *P<0.05, **P<0.001; ANOVA,n=3 independent experiments. On an average, 11–20 cells per condition were examined. (c) APP/APLP dKO cells were transfected with either wild-type G-PS1-R probe or G-PS1-R with FAD L166P mutation, and PS1 NT (GFP) to PS1-loop (RFP) proximity was analysed by FLIM (mean±s.d.; *P<0.05, ANOVA,n=3 independent experiments). On an average, 18–21 cells per condition were examined. (d) FLIM analysis of PS1 conformation in APP/APLP dKO cells co-transfected with G-PS1-R probe, together with either wild-type Pen-2 or N-terminally modified Flag-Pen-2 (mean±s.d.; *P<0.05, ANOVA,n=3 independent experiments). On an average, 14–16 cells per condition were examined. Figure 3: FLIM analysis of the changes in GFP-PS1-RFP conformation in APP/APLP2 dKO cells. ( a ) Schematic representation of the helical peptide, HP and GSM binding site on APP C99. ( b ) GSMs affect PS1 conformation (NT-loop proximity) in the presence of HP. APP/APLP dKO cells transfected with G-PS1-R probe were treated with either HP alone or HP together with fenofibrate (ff) or ibuprofen (ibu). The graph shows mean±s.d. lifetime in picoseconds; * P <0.05, ** P <0.001; ANOVA, n =3 independent experiments. On an average, 11–20 cells per condition were examined. ( c ) APP/APLP dKO cells were transfected with either wild-type G-PS1-R probe or G-PS1-R with FAD L166P mutation, and PS1 NT (GFP) to PS1-loop (RFP) proximity was analysed by FLIM (mean±s.d. ; * P <0.05, ANOVA, n =3 independent experiments). On an average, 18–21 cells per condition were examined. ( d ) FLIM analysis of PS1 conformation in APP/APLP dKO cells co-transfected with G-PS1-R probe, together with either wild-type Pen-2 or N-terminally modified Flag-Pen-2 (mean±s.d. ; * P <0.05, ANOVA, n =3 independent experiments). On an average, 14–16 cells per condition were examined. Full size image Manipulations of γ-secretase components change PS1 conformation We have previously shown that direct manipulation of γ-secretase components such as introduction of FAD linked mutations in PS1 [10] and modification of the Pen-2 NT [13] lead to a 'closed' conformation in APP-expressing cells. We asked whether, similar to GSMs, these conformational changes required the binding of substrate to the docking site. To test this, either G-PS1-R or G-PS1-R with the FAD-linked L166P mutation was transfected into APP/APLP dKO cells and NT-loop proximity was measured by FLIM. The lifetime of the GFP donor at the PS1 NT was shorter in the presence of the L166P mutation compared with that in the wild-type G-PS1-R ( Fig. 3c ). Similarly, co-transfection of G-PS1-R with wild-type Pen-2 or Pen-2 in which the NT is modified by addition of a Flag epitope tag [13] caused an alteration in PS1 conformation in Pen-2-flag-expressing APP/APLP2 dKO cells by bringing PS1 NT and the loop closer together, compared with that in cells expressing wild-type Pen-2 ( Fig. 3d ). Collectively, these results suggest that direct manipulations of these γ-secretase components affect PS1 conformation independently of the presence of APP/APLP2 substrates. Of note, overexpression of wild-type Pen-2, together with G-PS1-R, in APP/APLP2 cells leads to increased GFP lifetime compared with that in cells transfected with G-PS1-R alone, suggesting that, in the absence of APP substrate, Pen-2 expression causes 'opening' of the PS1 conformation. For comparison of different PS1 conformational states in APP/APLP2 dKO cells, we calculated the percentage of FRET efficiency for the G-PS1-R probe in different experimental conditions ( Supplementary Table S1 ). Given the substrate labelling by photoactivatable GSMs demonstrated by Kukar et al ., [8] we considered three possible mechanisms of action of GSMs. Perhaps the most straightforward explanation is that the binding of GSMs to APP leads to a change in how APP is presented to the γ-secretase catalytic site. Indeed, during preparation of this paper, another group presented data suggesting that binding of GSMs to the Aβ domain could affect the APP dimerization state, thereby altering the Aβ 42/40 ratio [21] . Alternatively, GSM-bound APP induces a change in PS1/γ-secretase conformation, which in turn alters the presentation of APP to the γ-secretase active site. This possibility is supported by our previous observation that the FAD-causing mutations in APP led to changes in PS1/γ-secretase conformation [22] . A more likely scenario is that the GSM binding site is on γ-secretase, close to the PS1/substrate interface, and that crosslinking to APP described by Kukar et al . [8] reveals this proximity. The first and second hypotheses cannot clearly explain our findings that, in the absence of APP, an HP, which lacks the putative GSM binding site, was quite unexpectedly able to mediate the effects of GSMs on PS1 conformation ( Fig. 3b ). In addition, Kukar et al . [8] reported that binding of GSMs to Notch is far less efficient than binding to APP, whereas in the current study fenofibrate and ibuprofen could modify PS1 conformation in the presence of Notch substrate, arguing against the 'substrate targeting' of GSMs. The substrate targeting of GSMs has been recently brought into question by a study demonstrating that mutations in the proposed GSM binding site on APP did not change the effect of GSMs on the Aβ 42/40 ratio [23] . Moreover, the specificity of GSMs binding to APP was challenged by an NMR-based study [24] . Furthermore, some aggressive PS1 mutations are resistant to the ability of NSAIDs to reduce the Aβ 42/40 ratio [25] . It is possible that as the 'closed' conformation of FAD-mutant PS1 is determined by the intrinsic molecular structure derived from its primary amino acid sequence, which forces PS1 into the 'closed' conformation, it may disable the access of GSMs to the allosteric site to a variable degree. Conversely, the Aβ 42 -raising APP mutants respond to GSMs that can reduce the Aβ 42 production as efficiently as the wild-type APP [23] , supporting the idea that GSMs function on the PS1/γ-secretase. Accordingly, direct manipulation of the potential GSM targets in the γ-secretase complex, either Pen-2 or PS1, causes conformational changes in PS1 even in the absence of APP/APLP2. On the basis of our findings, we propose a model for the action of GSMs on PS1 conformation ( Fig. 4 ). In this model, a hidden 'allosteric' site, presumably within the γ-secretase complex or at the PS1/substrate interface, becomes accessible to GSMs only after binding of the γ-secretase substrate or HP to a 'substrate docking site' (first step). Subsequent action of GSMs on the 'allosteric site' induces a PS1 conformational change (second step), which changes its alignment with the APP substrate and thus the site of γ-cleavage on APP. This model does not rule out the possibility that some GSMs may initially bind to the APP substrate or even to the HP used in this study. In this alternative scenario, binding of the APP transmembrane domain to the substrate-docking site on γ-secretase, which 'activates' the allosteric site, allows substrate-bound GSMs to exert an effect on the allosteric site located near the PS1/substrate interface to induce PS1 conformational change. In either scenario, our data suggest that substrate docking has a key role in mediating the effects of GSMs on PS1 conformation in intact cells, and the modulatory effect of GSMs is implemented through the 'allosteric site' apparently located within the γ-secretase complex. 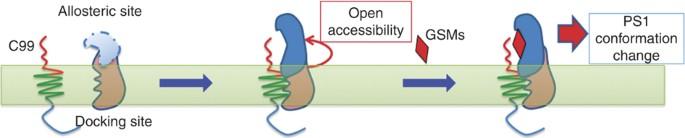Figure 4: Two-step model of the GSM action. The allosteric site responsible for PS1 conformational change and located within the γ-secretase complex is hidden in the absence of APP C99/NotchΔEC substrate. On binding of the substrate to the docking site, the allosteric site is 'activated' and becomes accessible for GSMs. Subsequent action of GSMs on the γ-secretase allosteric site leads to 'opening' or 'closing' of PS1 conformation. Figure 4: Two-step model of the GSM action. The allosteric site responsible for PS1 conformational change and located within the γ-secretase complex is hidden in the absence of APP C99/NotchΔEC substrate. On binding of the substrate to the docking site, the allosteric site is 'activated' and becomes accessible for GSMs. Subsequent action of GSMs on the γ-secretase allosteric site leads to 'opening' or 'closing' of PS1 conformation. Full size image Collectively, our report demonstrates that there are substrate-dependent and -independent factors underlying PS1 conformational changes after. We show that the transmembrane domain of the γ-secretase substrate has a significant role in enabling some GSMs (specifically fenofibrate, celcoxib, flurbiprofen and ibuprofen, used in this study) to induce conformational changes in PS1. It is plausible that numerous environmental factors could affect either APP substrate or PS1/γ-secretase directly to modulate the Aβ 42/40 ratio, and lead to pathological changes associated with AD. Thus, further understanding of the substrate-dependent and -independent effects on PS1 conformation and the Aβ 42/40 ratio is important for the design of therapeutic treatments. Cell lines and pharmacological treatments Mouse embryonal fibroblasts were obtained from APP/APLP2 −/− embryos and immortalized with a lentivirus expressing the SV40 T antigen without antibiotic selection. Following transformation, pooled mouse embryonal fibroblasts were stored for later use or subsequently stably transfected with FL human APP 695 complementary DNA through lentiviral infection and selected with hygromycin. All the transformants were used as pooled cultures without clonal selection. All protocols related to the use of animals were previously approved by the Institutional Animal Care and Use committee to ensure compliance with Federal, State and local government regulations and animal welfare organization guidelines. CHO cells were obtained from American Type Culture Collection. CHO cells stably expressing wild-type human APP 751 (7W cells) were described previously [17] . All cells were maintained in Opti-MEM (Invitrogen) supplemented with 5% fetal bovine serum. The cells were plated into four-chamber slides, transfected with various constructs and used for FLIM analyses. To evaluate the effect of GSMs on PS1 conformation, the cells were treated for 24 h with 100 μM fenofibrate (Sigma), 400 μM ibuprofen (Sigma), 375 μM fluibiprofen (Sigma), 10 μM celecoxib (Sigma), 400 μM Naproxen (Biomol) and 500 μM Aspirin (Fluka). Ethanol or DMSO was used as a vehicle control for GSM experiments. To analyse the effect of fenofibrate on the Aβ 42/40 ratio and G-PS1-R conformation, 7W cells were plated into 35 mm glass-bottomed dishes (Mat Tek) and treated with designated concentrations of fenofibrate for 24 h. The cells were subjected to FLIM assay, whereas the media were collected for human Aβ enzyme-linked immunosorbent assay (ELISA) to determine the Aβ 42/40 ratio. To compete out APP binding to the PS1/γ-secretase, cells were treated for 24 h with 100 nM HP (Boc-Val Gly Aib Val Val Ile Aib Phe Val-Aib OMe), which was designed to mimic a portion of the APP transmembrane domain [12] . To inhibit catalytic activity of the γ-secretase, 7W cells were treated for 24 h with either 1 μM WPE-III-31C [26] or 7.5 μM L685458 [27] (Sigma) transition state analogue inhibitors. Dimethylsulphoxide was used as a vehicle control for the inhibitor treatments. Constructs and transfections The generation of G-PS1-R and PS1-loop-RFP constructs was previously described [11] . C99, an APP C-terminal fragment construct, containing APP signal peptide (SP) was produced as follows: SP from APP was cloned into Nhe I– Hin dIII sites of the pcDNA 3.1 expression vector (Invitrogen). C99 sequence was amplified by PCR and cloned into Hin dIII– Kpn I sites of SP-pcDNA3.1. The amino acids between SP and C99 were mutated into DA (Asp-Ala) by site-directed mutagenesis [28] . N-terminally truncated Notch 1 receptor construct (NotchΔEC), which does not require ligand binding and represents a constitutively active immediate substrate for the γ-secretase, was a gift from Dr R. Kopan [29] . Human APP 695 tagged with GFP at its C terminus was produced as previously described [30] . Pen2 construct tagged with Flag on its NT was a gift from Dr Selkoe (BWH, Boston, MA). Expression plasmid for CLAC-P was a gift from Dr Takeshi Iwatsubo (Tokyo University, Japan) [20] . The constructs were transiently transfected into cells using Lipofectamine 2000 reagent (Invitrogen), according to the manufacturer's instructions. Western blot analysis For western blot analysis, cells plated into 35 mm cell culture dishes were lysed in buffer containing 1% CHAPSO (3-[(3-cholamidopropyl) dimethylammonio]-2-hydroxy-1-propanesulfonate), and the lysates were resolved on a 4–20% Tris-Glycin gel. Rabbit anti-APP C terminus (1:5,000, Sigma) and mouse anti-actin (1:10,000, Abcam) antibodies were used for the detection. ELISA The 7W cells cultured in 35 mm dishes were treated with designated concentrations of fenofibrate for 24 h. The conditioned medium was subjected to ELISA using a human β-amyloid (1–40 and 1–42) ELISA kit (WAKO), according to the manufacturer's instruction. FLIM The proximity between the PS1 NT and TM6-7 loop domain as an indicator of PS1 conformation was monitored by FLIM assay in live cells expressing G-PS1-R construct as previously described [11] . The GFP-PS1 construct, in which GFP donor lifetime is measured in the absence of an acceptor (FRET absent), was used as a negative control to determine baseline GFP lifetime. When RFP acceptor fluorophore is present within <10 nm proximity of the donor fluorophore, the GFP donor fluorophore lifetime shortens because of non-radiative transfer of a part of its emission energy to the RFP acceptor (FRET present). Thus, decrease in the GFP donor lifetime in the G-PS1-R construct indicates close proximity (<10 nm) between GFP fused to the PS1 NT and RFP fused into the PS1 loop domain. The degree of GFP lifetime shortening reflects proximity between GFP- and RFP-labelled epitopes, and serves as an indicator of G-PS1-R conformational changes. To analyse the effect of HP on APP–PS1 interactions in 7W cells, 7W cells were transiently co-transfected with APP-GFP- and PS1-RFP-expressing plasmids. The transfected cells were treated with either HP or transition state analogue inhibitors for 24 h and subjected to FLIM analysis. Cells were imaged on a Zeiss LCM510 microscope equipped with a 37 °C heating chamber containing 5% CO 2 . A Chameleon pulsed laser was used to excite GFP donor fluorophore (two-photon excitation wavelength at 840 nm). Becker&Hickl FLIM hardware and software (Becker&Hickl) were used to acquire the donor lifetime information. Data analysis was performed using SPC Image (Becker&Hickl), in which donor fluorophore lifetimes are determined by fitting the data to one (negative control) or two (experimental conditions) exponential decay curves, using whole cell as a region of interest. In the two-exponential model of lifetime analysis, the longer (no-FRET) lifetime is 'fixed' as a t 1 value, and the second, shorter lifetime reflecting the presence of FRET is calculated by the system as a t 2 value. The t 2 lifetime is used for comparisons between different experimental conditions. Thus, 'non-FRETing' component ( t 1, mainly perinuclear PS1 molecules that represent inactive PS1 holoprotein [10] ) is excluded from the lifetime comparisons. The donor lifetime information could be colour coded and displayed in a 128×128 pixel matrix as pseudo-colour images [10] . Statistical analysis StatView for Windows, version 5.0.1 (SAS Institute) was used to perform statistical analysis using Fisher's protected least significant difference analysis of variance (ANOVA). Samples were considered significantly different at P <0.05. How to cite this article: Uemura, K. et al . Substrate docking to γ-secretase allows access of γ-secretase modulators to an allosteric site. Nat. Commun. 1:130 doi: 10.1038/ncomms1129 (2010).